Metabolic learning and memory formation by the brain influence systemic metabolic homeostasis Metabolic homeostasis is regulated by the brain, but whether this regulation involves learning and memory of metabolic information remains unexplored. Here we use a calorie-based, taste-independent learning/memory paradigm to show that Drosophila form metabolic memories that help in balancing food choice with caloric intake; however, this metabolic learning or memory is lost under chronic high-calorie feeding. We show that loss of individual learning/memory-regulating genes causes a metabolic learning defect, leading to elevated trehalose and lipid levels. Importantly, this function of metabolic learning requires not only the mushroom body but also the hypothalamus-like pars intercerebralis, while NF-κB activation in the pars intercerebralis mimics chronic overnutrition in that it causes metabolic learning impairment and disorders. Finally, we evaluate this concept of metabolic learning/memory in mice, suggesting that the hypothalamus is involved in a form of nutritional learning and memory, which is critical for determining resistance or susceptibility to obesity. In conclusion, our data indicate that the brain, and potentially the hypothalamus, direct metabolic learning and the formation of memories, which contribute to the control of systemic metabolic homeostasis. Learning and memory formation are fundamental biological processes contributing to the survival of a species under changing environmental conditions. The brain is crucial for this function that is built up classically through processing the information from visual, auditory, olfactory, taste and other sensory systems. Compared with this traditional view on learning and memory, it is, however, unknown whether the central control of metabolic homeostasis chronically involves a form of learning and memorizing post-ingestive metabolic information independent of the sensory properties of food, which we briefly refer to as ‘metabolic learning/memory’. Of interest, recent research showed that flies can distinguish the nutritional value from the taste of food [1] , [2] ; however, questions remain regarding whether the brain can employ a mechanism of metabolic learning to regulate metabolic homeostasis and, if so, whether this function requires the brain region that critically mediates nutrient sensing, for example, the hypothalamus in mammals and pars intercerebralis (PI) in Drosophila . Moreover, from a disease perspective, it is worth exploring whether metabolic learning impairment mediates the development of metabolic diseases, especially since learning and memory disorders are often seen in overnutrition-induced diseases [3] . Here we developed a series of Drosophila and mouse models and obtained a body of results collectively suggesting that metabolic learning and memory formation by the brain, and potentially by the hypothalamus, is important for the central control of metabolic homeostasis, and dysfunction of this mechanism contributes to the development of metabolic diseases. Feeding control via metabolic learning in Drosophila In this work, we developed a Drosophila conditioning learning and memory paradigm, based on a literature-established taste/smell-matched food recipe using the same yeast content but altered sorbitol content, which provides an alternative but tasteless carbohydrate source [1] , [2] . An olfactory conditioning paradigm was used ( Supplementary Fig. 1 ), in which volatile chemicals 3-Octanol (OCT) and 4-Methylcyclohexanol (MCH) were used as conditional stimuli, a well-established approach in the literature [4] , while unconditional stimulus was a normal-calorie food (NC) containing 50 g l −1 sorbitol versus a high-calorie food (HC) containing 200 g l −1 sorbitol, both of which had the same yeast content (50 g l −1 ). Indeed, whether fed or fasting condition was tested, untrained Canton-S ( CS ) flies did not show any bias towards NC or HC when initially exposed to these two food types ( Supplementary Fig. 2a ), supporting that NC and HC had the same taste. Flies were trained to develop a learning/memory association between an odour and a food type. As elucidated in Supplementary Fig. 1 , for each training cycle, flies were kept 24 h in NC-containing vials circulated with one odour, and then 24 h in HC-containing vials circulated with the other odour. After a designated number of training cycles, flies were tested for conditional preference between two odours in the absence of food, in which flies were loaded at the middle joint section ( Supplementary Fig. 1 ) and their choices of OCT versus MCH vials were recorded. This conditional preference was reflected by Preference Index, calculated as ([number of flies that travelled to vials with NC-associated odour]—[number of flies that travelled to vials with HC-associated odour])/[total number of flies in both vials]. Results showed that following three to six training cycles, flies established a strong preference for NC-associated odour but a strong discrimination against HC-associated odour ( Fig. 1a,b ). In addition, we alternated these two odours in association with NC versus HC, and confirmed that flies always developed a preference to NC-associated odour whether MCH or OCT was matched ( Supplementary Fig. 2b ). We also confirmed that the Preference Index was not affected whether the flies were initially placed to NC or HC ( Supplementary Fig. 2c ). In addition, we considered that the training course was associated with age increase, and thus tested whether this age increase could have an impact on odour preference. To do so, we compared untrained flies at the ages matched with the flies prior to versus post training, and verified that this age increase per se did not lead to a bias for an odour ( Supplementary Fig. 2d ). Finally, to additionally evaluate this finding, we compared NC with a range of food sorbitol contents, including a low concentration (20 g l −1 ) and an extreme high concentration (300 g l −1 ) while the yeast content was the same (50 g l −1 ). We found that flies consistently preferred for NC-associated odour while being discriminated against HC or low-calorie food ( Fig. 1a ). Using food intake as a readout measurement, we observed that while untrained flies ate NC and HC similarly at cycle 0, they volunteered to eat a less amount of HC than NC after three to six training cycles ( Fig. 1c ). Taken together, these findings indicate that flies employ metabolic learning to form metabolic memory and thus decrease the exposure to overnutritional environment when normal nutritional environment is available. 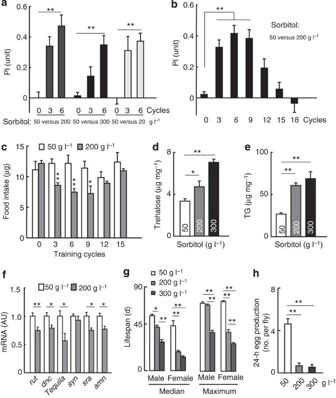Figure 1: Food and metabolic control via metabolic learning and memory formation. (a) AdultCSflies received the indicated training cycles in associating conditioned odour stimuli with NC (50 g l−1sorbitol) food versus a HC (200 or 300 g l−1sorbitol) or a low-calorie (20 g l−1sorbitol) food, and were tested for measuring the Preference Index (PI).n=60–80 animals per sample andn=4–8 samples per group. (b,c) AdultCSflies received the indicated training cycles in associating conditioned odour stimuli with NC (50 g l−1sorbitol) versus HC (200 g l−1sorbitol) food, and were subjected to the test for the PI (b) or measured for 30-min food intake (c).n=60–80 (b) or 10 (c) animals per sample, andn=4–8 samples per group. (d,e) AdultCSflies were maintained on NC (50 g l−1sorbitol) versus HC (200 or 300 g l−1sorbitol) food for 3 weeks. These flies were determined for body’s contents of trehalose (d) and TG (e).n=5 animals per sample andn=4–6 samples per group. (f) AdultCSflies were treated with NC (50 g l−1sorbitol) versus HC (200 g l−1sorbitol) food for 3 weeks. The mRNA levels of indicated learning/memory genes were determined. AU: arbitrary unit.n=15 animals per sample andn=5–6 samples per group. (g,h) AdultCSflies were maintained on NC (50 g l−1sorbitol) versus HC (200 or 300 g l−1sorbitol) food. These flies were determined for lifespan (g) and fecundity (h). (g) Lifespan assay was performed using Kaplan–Meier survival analysis, andPvalues were determined by log-rank test. Maximum lifespan analysis was conducted on the longest-lived 10% of flies in each group.n=30 (g) and 5 (h) animals per sample, andn=3 (g) and 12 (h) samples per group. **P<0.01, *P<0.05 ((a,b,d–h) analysis of variance (ANOVA) and Tukey; (c,f) unpaired Student’st-test); error bars reflect means±s.e.m. Figure 1: Food and metabolic control via metabolic learning and memory formation. ( a ) Adult CS flies received the indicated training cycles in associating conditioned odour stimuli with NC (50 g l −1 sorbitol) food versus a HC (200 or 300 g l −1 sorbitol) or a low-calorie (20 g l −1 sorbitol) food, and were tested for measuring the Preference Index (PI). n =60–80 animals per sample and n =4–8 samples per group. ( b , c ) Adult CS flies received the indicated training cycles in associating conditioned odour stimuli with NC (50 g l −1 sorbitol) versus HC (200 g l −1 sorbitol) food, and were subjected to the test for the PI ( b ) or measured for 30-min food intake ( c ). n =60–80 ( b ) or 10 ( c ) animals per sample, and n =4–8 samples per group. ( d , e ) Adult CS flies were maintained on NC (50 g l −1 sorbitol) versus HC (200 or 300 g l −1 sorbitol) food for 3 weeks. These flies were determined for body’s contents of trehalose ( d ) and TG ( e ). n =5 animals per sample and n =4–6 samples per group. ( f ) Adult CS flies were treated with NC (50 g l −1 sorbitol) versus HC (200 g l −1 sorbitol) food for 3 weeks. The mRNA levels of indicated learning/memory genes were determined. AU: arbitrary unit. n =15 animals per sample and n =5–6 samples per group. ( g , h ) Adult CS flies were maintained on NC (50 g l −1 sorbitol) versus HC (200 or 300 g l −1 sorbitol) food. These flies were determined for lifespan ( g ) and fecundity ( h ). ( g ) Lifespan assay was performed using Kaplan–Meier survival analysis, and P values were determined by log-rank test. Maximum lifespan analysis was conducted on the longest-lived 10% of flies in each group. n =30 ( g ) and 5 ( h ) animals per sample, and n =3 ( g ) and 12 ( h ) samples per group. ** P <0.01, * P <0.05 (( a , b , d – h ) analysis of variance (ANOVA) and Tukey; ( c , f ) unpaired Student’s t -test); error bars reflect means±s.e.m. Full size image Impaired metabolic learning/memory by chronic overnutrition As learning and memory disorders are often displayed in chronic overnutrition-induced diseases [3] , we were curious whether this relationship might apply to metabolic learning and memory formation. To test this idea, we subjected flies to a prolonged training course (up to 21 training cycles) and thus introduced a long-duration, although intermittent, HC feeding in this behavioural test. As shown in Fig. 1b , flies decreased their preference to NC after 12 training cycles that involved 12-day exposure to HC, and barely distinguished NC versus HC following 15–18 training cycles that involved a longer period of HC exposure. Following this finding, we asked whether the age increase during this training might contribute to metabolic learning impairment. To answer this question, we tested flies at an age that was matched with 18 training cycles shown in Fig. 1b ; however, they received only six training cycles before the Preference Index measurement. As shown in Supplementary Fig. 3 , these flies still showed a strong level of metabolic learning after six training cycles, indicating that the age increase during the training did not have an influence on learning and memory. We also measured food intake, showing that, while flies ate a less amount of HC than NC during 3–9 training cycles, this difference between two diets disappeared after 12–15 training cycles ( Fig. 1c ). Altogether, chronic exposure to overnutritional environment has an effect in impairing metabolic learning, pretty much like the scenario in which chronic overnutrition leads to learning and memory disorders as appreciated in the literature [3] . Next, since impaired metabolic learning was associated with increased high-caloric intake ( Fig. 1c ), we wanted to determine whether this increase in dietary caloric intake on a chronic basis could have a negative effect on metabolic physiology. To do so, we measured trehalose, a glucose disaccharide synthesized from intracellular glucose in the fat body, which is then secreted into the haemolymph. Indeed, increases in sorbitol content in the food led to increased trehalose levels in the body in a dose-dependent manner ( Fig. 1d ), and these increases in the body were consistent with increased trehalose levels in the haemolymph ( Supplementary Fig. 4 ). In addition consistently, increases in sorbitol content in the food led to a dose-dependent increase in triglyceride (TG) levels in the body ( Fig. 1e ). Hence, these flies developed hyperglycaemia and hyperlipidaemia, which collectively resemble diabetic or pre-diabetic changes in mammals under chronic overnutrition. Moreover, as shown in Fig. 1f , we consistently found that chronic treatment of high-sorbitol food led to downregulation of many learning/memory-regulating genes in the brain, including rutabaga ( rut) , dunce (dnc), tequila, sarah (sra), syndrome (syn) and amnesiac ( amn) , all of which are known to be important for learning and memory formation in Drosophila [5] , [6] , [7] , [8] . Finally, on the basis of the manifestation of diabetic and lipid disorders in these flies, the general health of these animals should be predicted to decline substantially; indeed, when maintained on this high-sorbitol food, these flies displayed lifespan shortening ( Fig. 1g ) and poor fecundity ( Fig. 1h ). This long-term compromise in health was at least an outcome of joint effects from metabolic learning defect and other independent mechanisms induced by chronic overnutrition. In summary, impaired metabolic learning and memory formation under chronic overnutrition have a negative impact on physiology and health. Requirement of rut gene in metabolic learning/memory Learning and memory formation has short-term and long-term forms, and according to the literature [8] , [9] , [10] , short-term learning and memory in the brain is importantly mediated by the rut gene, which encodes a type I adenylyl cyclase that functions to associate unconditional with conditional stimuli. It has been documented that rut is expressed only in a few brain regions, in particular, the mushroom body (MB) [11] . Using in situ hybridization, we confirmed that rut was expressed predominantly in the MB, while its expression in the PI was also appreciable ( Fig. 2a ). Supported by this background information, we decided to explore whether a mutation of this gene could affect metabolic learning. To do so, we studied whether metabolic learning could be affected by a rut mutation in a Drosophila mutant strain rut 2080 , which was reported to have impaired short-term learning [12] , [13] , [14] . Technically, rut 2080 flies have normal visual [14] , olfactory [15] and gustatory [16] functions, and were therefore suitable for the conditional training paradigm in our study. We verified that rut 2080 mutant had normal climbing activities, reproductive function and egg viability when fed on a regular food ( Supplementary Fig. 5 ), again supporting that these animals are appropriate for our behavioural test. Under normal food conditions without training, rut 2080 mutants and wild-type ( wt ) controls showed similar food intake and body weight during a 3-week follow-up. In addition, when responding to normal- versus high-sorbitol food, they did not show an immediate preference to a food type ( Supplementary Fig. 6 ). Subsequently, these mutant and wt animals were subjected to the training demonstrated in Supplementary Fig. 1 . Data show that wt controls showed metabolic learning and memory formation at training cycle 7, but rut 2080 mutants failed to do so ( Fig. 2b–d ). The failure of developing metabolic learning in these mutants was also indicated according to food intake measurement, showing that unlike wt , which discriminated against high-sorbitol food following six training cycles ( Supplementary Fig. 7a ), rut 2080 did not have this response despite the same training ( Supplementary Fig. 7b ). Accordingly, compared with wt controls, rut 2080 showed significant increases in trehalose and TG contents over this training course ( Fig. 2e,f ). Altogether, these data suggest that the rut gene is required in the formation of metabolic learning and memory formation. 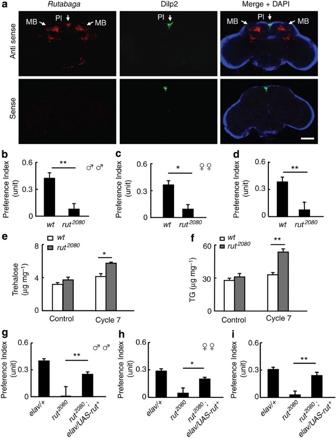Figure 2: Requirement of therutgene in metabolic learning and memory formation. (a) Adult brains ofCSflies were subjected toin situhybridization forrutabagamRNA (red) and immunostaining fordilp2antibody (green). Arrows point to the MB and the pars intercerebralis (PI) in the brain. Green fluorescence indicated the PI and was merged with red staining to showrutabagamRNA in this region. DAPI staining (blue) revealed the brain in this staining. Control group was stained with the sense mRNA probe and showed the absence of red staining. Scale bar, 100 μm. (b–f)rut2080flies andwild-type(wt) controls received seven cycles of training in olfactory conditioning test, and were analysed for Preference Index value (b–d) according to males (b), females (c) and both (d), and measured for body’s contents of trehalose (e) and TG (f). Basal controls were included on the basis of the matched flies that were fed on the same NC diet for the same training duration (e,f).n=60–80 (b–d) or 5 (e,f) animals per sample, andn=4–6 samples per group. (g–i) Flies includingrut2080,rut2080;elav-GAL4/UAS-rut+and controlelav-GAL4/+received seven cycles of training in olfactory conditioning test and analysed for Preference Index (g–i) according to males (g), females (h) and both genders (i).n=50–70 animals per sample, andn=4–6 samples per group. **P<0.01, *P<0.05 ((b–d) unpaired Student’st-test; (e–i) ANOVA and Tukey); error bars reflect means±s.e.m. Figure 2: Requirement of the rut gene in metabolic learning and memory formation. ( a ) Adult brains of CS flies were subjected to in situ hybridization for rutabaga mRNA (red) and immunostaining for dilp2 antibody (green). Arrows point to the MB and the pars intercerebralis (PI) in the brain. Green fluorescence indicated the PI and was merged with red staining to show rutabaga mRNA in this region. DAPI staining (blue) revealed the brain in this staining. Control group was stained with the sense mRNA probe and showed the absence of red staining. Scale bar, 100 μm. ( b – f ) rut 2080 flies and wild-type ( wt ) controls received seven cycles of training in olfactory conditioning test, and were analysed for Preference Index value ( b – d ) according to males ( b ), females ( c ) and both ( d ), and measured for body’s contents of trehalose ( e ) and TG ( f ). Basal controls were included on the basis of the matched flies that were fed on the same NC diet for the same training duration ( e , f ). n =60–80 ( b – d ) or 5 ( e , f ) animals per sample, and n =4–6 samples per group. ( g – i ) Flies including rut 2080 , rut 2080 ; elav-GAL4/UAS-rut + and control elav-GAL4/+ received seven cycles of training in olfactory conditioning test and analysed for Preference Index ( g – i ) according to males ( g ), females ( h ) and both genders ( i ). n =50–70 animals per sample, and n =4–6 samples per group. ** P <0.01, * P <0.05 (( b – d ) unpaired Student’s t -test; ( e – i ) ANOVA and Tukey); error bars reflect means±s.e.m. Full size image To further address whether the neural system is important for the phenotype that we observed in rut 2080 , we restored the wild-type copy of the rut gene selectively in the neural system of rut 2080 . This restoration was achieved by crossing rut 2080 ;UAS-rut + flies [12] , [13] , [14] , [17] to flies that expressed GAL4 under the control of a pan-neural elav promoter. Progenies, which had neuronal rut + expression due to GAL4 -induced UAS activation, were collected and analysed to determine whether a rescue effect could be achieved. Data revealed that restoration of rut in the neural system led to a significant reversal of metabolic learning defect in rut 2080 mutants ( Fig. 2g–i ). Moreover, this neural restoration of rut significantly protected against trehalose and TG increases in rut 2080 mutants ( Supplementary Fig. 8 ). Hence, these data lend a support to the model that rut in the brain is important for metabolic learning and memory formation. Requirement of dnc and tequila in metabolic learning/memory In addition to rut , we studied several other learning/memory-regulating genes, including dnc and tequila , which are also important for learning and memory formation [6] , [7] , [18] , [19] , [20] , [21] , [22] . Regarding dnc , it encodes a phosphodiesterase enzyme that hydrolyses cAMP, and coordinates with the learning/memory-regulatory function of rut to maintain cAMP in a normal range for short-term memory [7] , [18] , [19] . In our study, we tested dunce 1 flies, a line of dnc mutant Drosophila established in the literature [20] , [21] . When fed on a regular food, we confirmed that dunce 1 had normal locomotion ( Supplementary Fig. 5a ), although female dunce 1 had lower reproductive activities ( Supplementary Fig. 5b,c ). Under normal conditions, untrained dunce 1 and wt flies showed similar food intake and body weight, and no immediate preference for food types was confirmed when exposed to normal- versus high-sorbitol food ( Supplementary Fig. 6 ). However, following training cycles, we found that just like rut 2080 , these mutant flies showed a loss of conditional preference for normal-sorbitol food compared with wt flies ( Fig. 3a–c ). In addition, unlike wt , which developed a discrimination against high-sorbitol food over six training cycles ( Supplementary Fig. 7a ), dunce 1 did not have this discrimination regardless of the same training ( Supplementary Fig. 7c ), and this effect was associated with increased trehalose and TG levels ( Fig. 3d,e ). In parallel with dnc , the tequila gene was studied as well, which encodes a neurotrypsin orthologue; on the basis of a tequila mutant line ( teq − ), this gene is known to be important for long-term memory [6] , [22] . After having confirmed the suitability of this fly model for our behavioural test ( Supplementary Figs 5 and 6 ), we subjected teq − and wt to the learning and memory training, and revealed that these mutants also showed a significant defect in metabolic learning ( Fig. 4a–c ), which was accompanied by metabolic disorders ( Fig. 4d,e ). In summary, multiple learning/memory-regulating genes are involved in metabolic learning and memory formation. 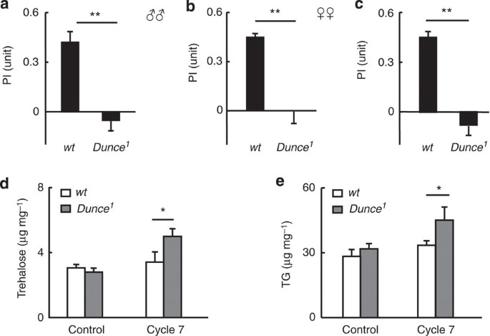Figure 3: Requirement of thedncgene in metabolic learning and memory formation. Dunce1andwtflies received seven cycles of training in olfactory conditioning test, and then were analysed for PI (a–c) according to males (a), females (b) and both (c), and measured for body’s contents of trehalose (d) and TG (e). Basal controls were included on the basis of separate groups of these flies that were fed on the same NC diet for the same training duration (d,e).n=50–70 (a–c) and 4–6 (d,e) animals per sample, andn=4–6 samples per group. **P<0.01, *P<0.05 ((a–c) unpaired Student’st-test; (d,e) ANOVA and Tukey); error bars reflect means±s.e.m. Figure 3: Requirement of the dnc gene in metabolic learning and memory formation. Dunce 1 and wt flies received seven cycles of training in olfactory conditioning test, and then were analysed for PI ( a – c ) according to males ( a ), females ( b ) and both ( c ), and measured for body’s contents of trehalose ( d ) and TG ( e ). Basal controls were included on the basis of separate groups of these flies that were fed on the same NC diet for the same training duration ( d , e ). n =50–70 ( a – c ) and 4–6 ( d , e ) animals per sample, and n =4–6 samples per group. ** P <0.01, * P <0.05 (( a – c ) unpaired Student’s t -test; ( d , e ) ANOVA and Tukey); error bars reflect means±s.e.m. 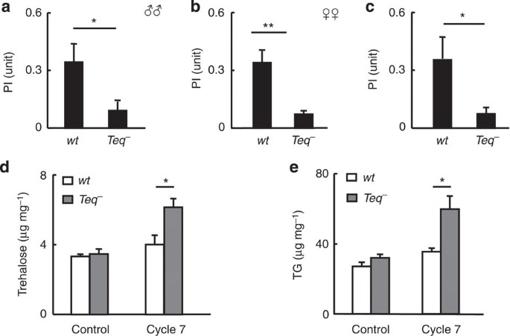Figure 4: Requirement of thetequilagene in metabolic learning and memory formation. Teq−andwtflies received seven cycles of training in olfactory conditioning test, and were analysed for PI (a–c) according to males (a), females (b) and both (c), and were measured for body’s contents of trehalose (d) and TG (e). Basal controls were included on the basis of separate groups of these flies that were fed on the same NC diet for the same training duration (d,e).n=50–70 (a–c) and 4–6 (d,e) animals per sample, andn=4–6 samples per group.**P<0.01, *P<0.05 ((a–c) unpaired Student’st-test; (d,e) ANOVA and Tukey); error bars reflect means±s.e.m. Full size image Figure 4: Requirement of the tequila gene in metabolic learning and memory formation. Teq − and wt flies received seven cycles of training in olfactory conditioning test, and were analysed for PI ( a – c ) according to males ( a ), females ( b ) and both ( c ), and were measured for body’s contents of trehalose ( d ) and TG ( e ). Basal controls were included on the basis of separate groups of these flies that were fed on the same NC diet for the same training duration ( d , e ). n =50–70 ( a – c ) and 4–6 ( d , e ) animals per sample, and n =4–6 samples per group. ** P <0.01, * P <0.05 (( a – c ) unpaired Student’s t -test; ( d , e ) ANOVA and Tukey); error bars reflect means±s.e.m. Full size image Requirement of the MB in metabolic learning/memory To understand the neuronal types that potentially convey metabolic information to a learning process, we first investigated neurons in the MB, a brain region that is classically known for inducing learning and memory in Drosophila [23] . As established, rut and dnc are two key genes that regulate cAMP balance in the MB, and disruption of each in the MB is sufficient to impair learning and memory formation [24] . Thus, to examine whether the MB neurons are required for metabolic learning, we employed an MB-specific GAL4 line ( 17D-GAL4 ) to inhibit the rut or dnc gene by crossing this GAL4 strain with either UAS-rut RNAi or UAS-dnc RNAi flies to create 17D-GAL4/UAS-rut RNAi and 17D-GAL4/UAS-dnc RNAi flies, respectively. As described in Methods, these UAS-RNAi strains were created using the VALIUM10 vector system, which is known to sufficiently induce RNA interference (RNAi) knockdown without additionally introducing dicer [25] . Our subsequent study revealed that both of these fly lines showed the absence of metabolic learning under training ( Fig. 5a,b ). In addition to these two fly models, we generated a third one in which we directly targeted PKA, a key component downstream of the protein encoded by rut , which is needed for the function of MB in inducing learning and memory [26] . To do so, we used inhibitory PKA (PKA inh ), which has a mutant cAMP-binding site and thus inhibits the function of rut in regulating learning and memory formation [27] . We therefore generated an MB-specific transgenic line with PKA inh expression by crossing 17D-GAL4 with UAS-PKA inh flies, resulting in 17D-GAL4/UAS-PKA inh flies. By examining these mutants, we found that PKA inhibition in this fly model led to a partial reduction in metabolic learning and memory formation ( Fig. 5c ). Finally, we profiled the metabolic physiology of these three fly models versus their controls, and results consistently demonstrated that the trehalose and TG levels in all these mutant animals significantly increased, although to different degrees ( Supplementary Fig 9a,b ). In summary, the MB is involved in mediating metabolic learning and memory formation in Drosophila . 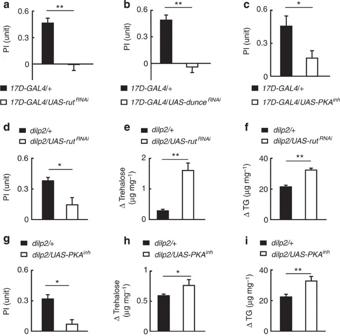Figure 5: The MB anddilp2-defined PI neurons in metabolic learning and memory formation. (a–c) Mutant flies including17D-GAL4/UAS-rutRNAi(a), 17D-GAL4/UAS-dunceRNAi(b),17D-GAL4/UAS-PKAinh(c) and matched controls17D-GAL4/+received six cycles of training, and then were analysed for PI.n=50–70 animals per sample, andn=4–6 samples per group. (d–i) Flies includingdilp2-GAL4/UAS-rutRNAi(shown asdilp2/UAS-rutRNAi) versus matched control groupdilp2-GAL4/+ (shown asdilp2/+) anddilp2-GAL4/UAS-PKAinh(shown asdilp2/UAS-PKAinh) versus matched control groupdilp2-GAL4/+ received 6–9 cycles of training, and then were analysed for PI (d,g) and body’s contents of trehalose (e,h) and TG (f,i). Data ine,f,h,ishowed the change levels (Δ) after training cycles compared with the levels of basal controls in which flies were maintained on the same NC diet for the same training duration.n=40–60 (d,g) or 5 (e,f,h,i) animals per sample, andn=4–6 samples per group. **P<0.01, *P<0.05 (unpaired Student’st-test); error bars reflect means±s.e.m. Figure 5: The MB and dilp2 -defined PI neurons in metabolic learning and memory formation. 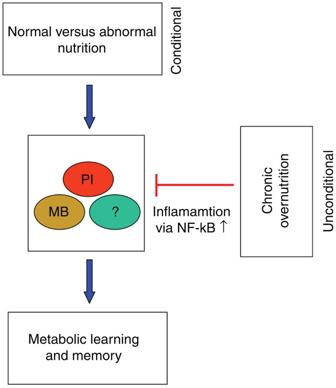Figure 9: Working model of metabolic learning and memory formation. Under an environmental condition containing normal and abnormal nutrition,Drosophilacan develop a form of learning and memory of metabolic information, referred to as ‘metabolic learning & memory’, to mediate the central control of metabolic homeostasis, which requires cooperative actions of the MB and PI neurons. However, chronic overnutrition can employ NF-κB-driven neuroinflammation to impair this form of learning and memory, contributing to the development of overnutrition-induced metabolic disorders and diseases. ( a–c ) Mutant flies including 17D-GAL4/UAS-rut RNAi ( a ) , 17D-GAL4/UAS-dunce RNAi ( b ), 17D-GAL4/UAS-PKA inh ( c ) and matched controls 17D-GAL4/+ received six cycles of training, and then were analysed for PI. n =50–70 animals per sample, and n =4–6 samples per group. ( d – i ) Flies including dilp2-GAL4/UAS-rut RNA i (shown as dilp2/UAS-rut RNA i ) versus matched control group dilp2-GAL4 /+ (shown as dilp2/+ ) and dilp2-GAL4 / UAS-PKA inh (shown as dilp2/UAS-PKA inh ) versus matched control group dilp2-GAL4 /+ received 6–9 cycles of training, and then were analysed for PI ( d , g ) and body’s contents of trehalose ( e , h ) and TG ( f , i ). Data in e , f , h , i showed the change levels (Δ) after training cycles compared with the levels of basal controls in which flies were maintained on the same NC diet for the same training duration. n =40–60 ( d , g ) or 5 ( e , f , h , i ) animals per sample, and n =4–6 samples per group. ** P <0.01, * P <0.05 (unpaired Student’s t -test); error bars reflect means±s.e.m. Full size image Requirement of the PI region in metabolic learning/memory Equivalent to mammalian hypothalamic neurons, Drosophila has a group of endocrine neurons in the hypothalamus-like PI region, which produce Drosophila insulin-like peptides (dilps) and have been genetically targeted in dilp2-GAL4 flies, which provide a Drosophila tool to study this neuronal population [28] , [29] , [30] , [31] . Indeed, defects in these dilp2-GAL4 -defined neurons can cause many metabolic disorders including diabetes and related diseases [30] , [31] . This knowledge led us to hypothesize that these dilp2 - GAL4 -defined PI neurons might participate in metabolic learning. To test this hypothesis, we inhibited rut in these neurons by crossing dilp2-GAL4 with UAS-rut RNAi flies to create dilp2-GAL4/UAS-rut RNAi flies. Using our training paradigm, we observed that these mutant flies showed poor function of metabolic learning ( Fig. 5d ). As a result of this defect, these mutant flies showed significant increases in trehalose and TG levels ( Fig. 5e,f ). To further evaluate the role of these neurons in metabolic learning and memory formation, we independently generated another fly model in which PKA inh was expressed specifically in dilp2-GAL4 -defined neurons. To do so, we crossed dilp2 -GAL4 with UAS-PKA inh to generate dilp2-GAL4/UAS-PKA inh flies. These mutant flies also demonstrated a defective function of metabolic learning ( Fig. 5g ) and increased levels in trehalose and TG ( Fig. 5h,i ) during the training course. These results suggest that dilp2-expressing neurons in the PI region are necessary for the process of metabolic learning. Admittedly, this study did not address whether the role of PI neurons in regulating metabolic learning is independent of the signalling of dilp2 and perhaps other dilps. Regardless, this possibility can be reasoned, considering that PKA was reported to negatively affect insulin/IGF signalling in flies [32] , and our results suggest that PKA in the dilp2 - GAL4 -defined neurons is needed for metabolic learning. Thus, future studies are needed to study whether dilps might participate in the function of PI in mediating metabolic learning. In summary, certain neurons in the PI work cooperatively with the MB to mediate metabolic learning and memory formation. Overnutrition impairs metabolic learning via inflammation Recently, using mouse models, we have established that chronic overnutrition induces NF-κB-dependent hypothalamic inflammation and causes obesity and diabetes [33] , [34] . In relation with this background, our studies in this work elucidated that metabolic learning not only requires the hypothalamus-like PI region but also can be impaired under chronic overnutrition. Thus, we logically asked whether the NF-κB-induced inflammatory pathway might link overnutrition to metabolic learning impairment in Drosophila . Regarding the NF-κB pathway, three NF-κB transcription factors have been identified in Drosophila , including dorsal ( dl) , disordered facets ( dif) and Relish ( Rel) , which represent the key regulators of immune response [35] . Results showed that, while chronic HC feeding decreased the expression of leaning/memory genes in flies (Fig. 1f), it increased the brain expression levels of NF-κB pathway components including dl , dif and Rel as well as many pro-inflammatory cytokine genes such as outstretched ( os) , unpaired 2 ( upd2) and eiger ( egr) (Fig. 6a ). Although we do not predict that these increases are responsible for NF-κB activation, these changes clearly indicate an inflammatory state that can reflect NF-κB activation. These effects of high-sorbitol feeding were specific to the brain, since the expression levels of these genes in the periphery of the body did not show significant changes ( Supplementary Fig. 10 ). Hence, these findings triggered us to question whether metabolic learning could be affected by NF-κB in the brain and, in particular, the PI in the brain. To answer this question, we generated a Drosophila model with neural NF-κB activation, by crossing elav-GAL4 with UAS-dl flies. Supportedly, data revealed that elav-GAL4/UAS-dl flies showed an impairment in metabolic learning and memory formation ( Fig. 6b ), and this defect was consistently associated with trehalose and lipid disorders ( Supplementary Fig. 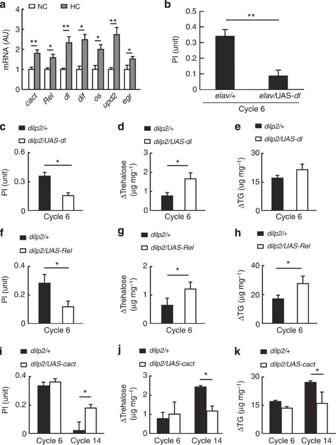11 ). Figure 6: Impairment of metabolic learning and memory formation by the NF-κB pathway. (a) Brain expression levels of inflammation-related genes in the adultCSflies after 18 days NC (50 g l−1) or HC (200 g l−1) food treatment. AU: arbitrary unit.n=30 animals per sample andn=4 samples per group. (b–k) Flieselav-GAL4/UAS-dl(shown aselav/UAS-dl) versus controlelav-GAL4/+(shown aselav/+) (b),dilp2-GAL4/UAS-dl(shown asdilp2/UAS-dl) versus controldilp2-GAL4/+ (c–e),dilp2-GAL4/UAS-Rel(shown asdilp2/UAS-Rel) versus controldilp2-GAL4/+ (f–h) anddilp2-GAL4/UAS-cact(shown asdilp2/UAS-cactversus controldilp2-GAL4/+ (i–k) received indicated cycles of training, and then were analysed for PI (b,c,f,i) and body’s contents of trehalose (d,g,j) and TG (e,h,k). Data in (d,e,g,h,j,k) showed the change levels (Δ) after indicated training cycles compared with the levels of basal controls in which flies were maintained on the same NC diet for the same training duration.n=50–70 (b,c,f,i) or 5 (d,e,g,h,j,k) animals per sample, andn=4–8 samples per group. **P<0.01, *P<0.05 ((a–h) unpaired Student’st-test; (i–k) ANOVA and Tukey); error bars reflect means±s.e.m. Figure 6: Impairment of metabolic learning and memory formation by the NF-κB pathway. ( a ) Brain expression levels of inflammation-related genes in the adult CS flies after 18 days NC (50 g l −1 ) or HC (200 g l −1 ) food treatment. AU: arbitrary unit. n =30 animals per sample and n =4 samples per group. ( b – k ) Flies elav-GAL4/UAS-dl (shown as elav/UAS-dl ) versus control elav-GAL4/+ (shown as elav/+ ) ( b ), dilp2-GAL4/UAS-dl (shown as dilp2/UAS-dl ) versus control dilp2-GAL4 /+ ( c – e ), dilp2-GAL4/UAS-Rel (shown as dilp2/UAS-Rel ) versus control dilp2-GAL4 /+ ( f – h ) and dilp2-GAL4/UAS-cact (shown as dilp2/UAS-cact versus control dilp2-GAL4 /+ ( i – k ) received indicated cycles of training, and then were analysed for PI ( b , c , f , i ) and body’s contents of trehalose ( d , g , j ) and TG ( e , h , k ). Data in ( d , e , g , h , j , k ) showed the change levels (Δ) after indicated training cycles compared with the levels of basal controls in which flies were maintained on the same NC diet for the same training duration. n =50–70 ( b , c , f , i ) or 5 ( d , e , g , h , j , k ) animals per sample, and n =4–8 samples per group. ** P <0.01, * P <0.05 (( a – h ) unpaired Student’s t -test; ( i – k ) ANOVA and Tukey); error bars reflect means±s.e.m. Full size image Next, we narrowed down to dilp2 - GAL4 -defined neurons in the PI, and thus generated two independent lines of NF-κB activation specifically in these neurons, through crossing dilp2-GAL4 flies with either UAS-dl or UAS-Rel flies, resulting in dilp2-GAL4/UAS-dl and dilp2-GAL4/UAS-Rel flies, respectively. These flies and their matched controls were examined using the training paradigm described above, and we found that both of these mutant lines showed impaired metabolic learning as well as increases in trehalose and TG levels ( Fig. 6c–h ), confirming that NF-κB in the PI region is a link between chronic overnutrition and its effect in impairing metabolic learning. Finally, we studied whether NF-κB inhibition in these PI neurons could offer a protective effect for improving metabolic learning and memory formation under chronic overnutrition. To do so, we created a fly model with dilp2 neuron-specific overexpression of cactus (cact) , since Cactus is homologous to vertebrate IκBα protein, which is a specific and potent inhibitor of NF-κB signalling [36] , [37] , [38] . This genetic model was created through crossing dilp2-GAL4 with UAS-cact flies and was subjected to a long-duration exposure to high-sorbitol food using a 4-week training course. As similarly observed in Fig. 1b , control flies showed a significant defect in metabolic learning and memory formation after 14 training cycles; in contrast, dilp2-GAL4/UAS-cact flies still maintained a good level of metabolic learning ( Fig. 6i ). In alignment with this protective effect, these mutant flies exhibited counteraction against overnutrition-induced trehalose and TG increases during this long training course ( Fig. 6j,k ). Taken together, activation of the NF-κB pathway in the brain and PI region in particular has a negative impact on metabolic learning and memory formation. Hypothalamic learning/memory genes in mice with obesity With great interest, we employed a mouse model to evaluate the potential involvement of the hypothalamus in metabolic learning. To do so, we designed a study in which A/J mice and C57BL/6J mice were compared because these two strains are resistant against and prone to dietary obesity, respectively [39] , and they have different nutritional preferences when subjected to free choice between high-fat and low-fat diets [40] , [41] . Specifically, we analysed these mice, in order to explore if the different metabolic responses between these two strains might be related to different brain programmes of learning and memory. In our experiment, our examination was focused on a list of learning/memory-regulating genes, including adenylate cyclase 8 ( Adcy8) , SH3/ankyrin domain gene 3 ( Shank3) , synaptosomal-associated protein 25 ( Snap25) , discs large homologue 3 and 4 ( Dlg3, 4) , calcium/calmodulin-dependent protein kinase II α, β and γ (Camk2a, b, g) and activity regulated cytoskeletal-associated protein (Arc) , each of which is important for learning and memory formation [42] , [43] , [44] , [45] , [46] , [47] , [48] . Indeed, we confirmed that these genes were highly expressed in the hippocampus of mice, but surprisingly, the hippocampal expression levels of these genes did not differ much between A/J and C57BL/6J mice ( Fig. 7a ). When the hypothalamus was analysed, a number of these genes were found to strongly express in the hypothalamus and, importantly, these genes were differentially expressed in the hypothalamus of A/J versus C57BL/6J mice. As shown in Fig. 7b , we found that Adcy8 , Snap25 and Camk2g were downregulated while Shank3 , Dlg4 and Arc were upregulated in the hypothalamus of C57BL/6J mice compared with A/J mice. Supported by this finding, we asked whether some of these changes could be induced in a separate mouse model that suffers from obesity development. We therefore employed chronic high-fat diet (HFD) feeding, since it is an important aetiological factor for dietary obesity and related metabolic disorders. Results showed that compared with normal chow-feeding, 3-month HFD feeding barely affected the hippocampal expression of these genes except Dlg4 ( Fig. 7c ), but broadly affected the expression of these genes including Adcy8 , Shank3 , Snap25 , Dlg3, Dlg4, Camk2b and Arc in the hypothalamus ( Fig. 7d ). By analogy, these HFD-induced hypothalamic changes significantly reflected the difference in the hypothalamus of A/J versus C57BL/6J mice. 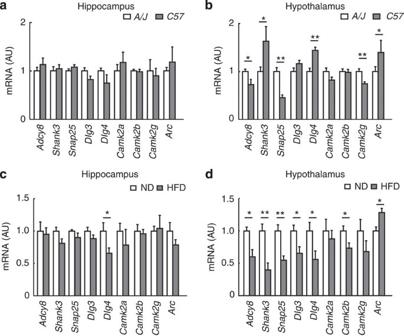These molecular lines of evidence provided a suggestion to the concept that the hypothalamus is involved in a form of learning and memory formation in regulating body weight control and affecting obesity development. Figure 7: Involvement of the hypothalamus in learning/memory-regulating genes of mice. (a,b) Hippocampal (a) and hypothalamic (b) levels of learning/memory genes inA/JandC57BL/6Jmice (∼3-month-old males) under basal and normal chow-feeding conditions. (c,d) The mRNA levels of learning/memory genes were determined for the hypothalamus (b) and hippocampus (c) of adult maleC57BL/6Jmice that received 3-month ND versus HFD feeding. **P<0.01, *P<0.05 (unpaired Student’st-test),n=4–6 mice per group; error bars reflect means±s.e.m. Figure 7: Involvement of the hypothalamus in learning/memory-regulating genes of mice. ( a , b ) Hippocampal ( a ) and hypothalamic ( b ) levels of learning/memory genes in A/J and C57BL/6J mice ( ∼ 3-month-old males) under basal and normal chow-feeding conditions. ( c , d ) The mRNA levels of learning/memory genes were determined for the hypothalamus ( b ) and hippocampus ( c ) of adult male C57BL/6J mice that received 3-month ND versus HFD feeding. ** P <0.01, * P <0.05 (unpaired Student’s t -test), n =4–6 mice per group; error bars reflect means±s.e.m. Full size image Nutritional learning/memory in mice with obesity resistance Following the molecular study presented above, we switched to physiological study in which a behavioural paradigm was used to test whether A/J and C57BL/6J mice have different learning and memory to distinguish normal versus HC food. First, these mice were examined via a visual cliff test, showing that A/J and C57BL/6J mice had the same safe responses ( A/J : 84.37±2.61% versus C57BL/6J : 83.13±3.43%). This result indicated that these two groups of animals had required vision for performing our behavioural test. Subsequently, using a modified method according to the literature [49] , [50] , [51] , [52] , we associated a green versus blue symbol with normal diet (ND, 10% kcal fat) versus HFD (45% kcal fat), two diets having the same colour (red), the same sucrose content and matched nutrient composition except for the fat to carbohydrate ratio. Mice were subjected to a training of learning and memory formation followed by measuring the Preference Index, as detailed in Methods. Data show that at the beginning of this training, A/J and C57BL/6J mice did not have an evident bias towards HFD or ND ( Fig. 8a,b ). However, by training cycle 6, A/J mice showed memory formation in favour of choosing ND, with this effect being maintained during training cycles 6–12 ( Fig. 8a ). Thus, despite HFD having a strong rewarding property [53] , this reward seemed to be over-ridden by a form of memory in A/J mice, although it was unclear whether ND-induced appetitive memory or HFD-induced aversive memory was accountable. On the other hand, we noted that over a long training course (15 cycles), this learning and memory function in A/J mice declined ( Fig. 8a ). We speculate that prolonged exposure to HFD led to an impairment in this form of memory, which weakened its counterbalance against HFD-induced reward. In contrast, throughout the training, C57BL/6J mice failed to establish this memory of favouring ND preference ( Fig. 8b ), implicating that this mouse strain has defects in generating this form of memory. In the meanwhile, HFD-induced reward response was clearly induced in C57BL/6J mice, as these animals showed a preference for HFD following three to six training cycles. 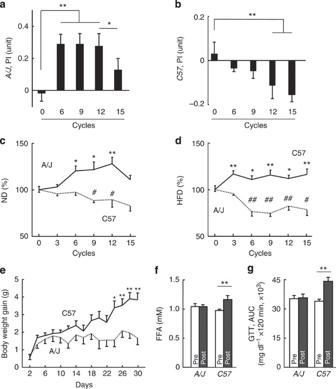Altogether, these results suggested that there might be a form of memory in mammals contributing to metabolic control in a manner that differs from the memory mechanism in HFD-promoted rewarding response. Figure 8: Different metabolic learning/memory profiles inA/JversusC57BL/6Jmice. (a,b) PI ofA/J(a) andC57BL/6J(b) mice following indicated training cycles. The PI was calculated as the time difference that mice spent in a cage of a conditioned stimulus associated with ND versus HFD divided by the total time. (c,d) Percentage changes of ND intake (c) versus HFD intake (d) inA/JandC57BL/6Jmice at the indicated training cycles relative to food intake at training cycle 0. Statistics reflect comparison with 0 cycle in each strain. (e) Body weight gain ofA/JandC57BL/6Jmice at the indicated days during the training. Statistics reflect comparisons betweenC57andA/Jat matched time points. (f) Serum FFA inC57BL/6JandA/Jbefore training (Pre) versus post 21 training cycles (Post). (g) Calculated values for area under curve (AUC) during 120-min glucose tolerance test ofA/JandC57BL/6Jmice before training (Pre) versus post 21 training cycles (Post).n=8–10 (a–e) andn=5–8 mice (f,g) per group. **P<0.01,##P<0.01, *P<0.05,#P<0.05 (ANOVA and Tukey); error bars reflect means±s.e.m. Figure 8: Different metabolic learning/memory profiles in A/J versus C57BL/6J mice. ( a , b ) PI of A/J ( a ) and C57BL/6J ( b ) mice following indicated training cycles. The PI was calculated as the time difference that mice spent in a cage of a conditioned stimulus associated with ND versus HFD divided by the total time. ( c , d ) Percentage changes of ND intake ( c ) versus HFD intake ( d ) in A/J and C57BL/6J mice at the indicated training cycles relative to food intake at training cycle 0. Statistics reflect comparison with 0 cycle in each strain. ( e ) Body weight gain of A/J and C57BL/6J mice at the indicated days during the training. Statistics reflect comparisons between C57 and A/J at matched time points. ( f ) Serum FFA in C57BL/6J and A/J before training (Pre) versus post 21 training cycles (Post). ( g ) Calculated values for area under curve (AUC) during 120-min glucose tolerance test of A/J and C57BL/6J mice before training (Pre) versus post 21 training cycles (Post). n =8–10 ( a – e ) and n =5–8 mice ( f , g ) per group. ** P <0.01, ## P <0.01, * P <0.05, # P <0.05 (ANOVA and Tukey); error bars reflect means±s.e.m. Full size image To explore whether this particular memory contributes to the control of metabolic physiology, we applied the same learning and memory training to A/J versus C57BL/6J mice and longitudinally profiled food intake and body weight gain in these mice. To control this experiment, we confirmed that these mice had comparable food intake under chow-feeding before training ( A/J : 3.40±0.48 g versus C57BL/6J : 3.71±0.26 g). Following three training cycles, A/J mice exhibited a gradual increase in ND intake ( Fig. 8c ) while a gradual decrease in HFD intake ( Fig. 8d ), resulting in increases in the ratio of ND to HFD intake. In contrast, C57BL/6J mice showed a gradual decrease in ND intake and an increase in HFD intake after three training cycles ( Fig. 8c,d ). Further, C57BL/6 mice displayed a greater degree of body weight gain compared with A/J mice following the completion of 12 training cycles ( Fig. 8e ). As a result of obesity resistance in A/J mice versus obesity susceptibility in C57BL/6J mice, these two strains showed phenotypic differences in light of obesity-associated metabolic disorders such as hyperlipidaemia and glucose intolerance. Before training, these two strains had comparable levels of circulating free fatty acids (FFA) ( Fig. 8f ) and comparable glucose tolerance ( Fig. 8g ). However, after 6 weeks of training, C57BL/6J mice showed increases in circulating free fatty acids ( Fig. 8f ) and glucose intolerance ( Fig. 8g ), which was clearly a result of HFD exposure during the training course. In contrast, A/J mice were protected from developing these metabolic disorders ( Fig. 8f,g ). In summary, these findings suggested that the central control of metabolic homeostasis probably involves a form of nutritional memory, which is dissociable from HFD reward-induced feeding response; however, the mechanism of forming this memory sensitively succumbs to the disruption under chronic overnutrition especially HFD feeding. In this work, we performed a series of studies in Drosophila and discovered that these animals temporarily develop metabolic learning to balance food choice with caloric intake. In Drosophila research, sugar has often been used for studying the appetitive reward value of food taste. Of interest, recent research has suggested that fruit flies can distinguish caloric values from the taste property of food [1] , [2] . Here using tasteless sorbitol as a carbohydrate source to generate an environmental condition that contained NC versus HC food, we revealed that Drosophila can develop a form of metabolic learning and memory independently of taste, by which flies are guided to have a preference for normal caloric environment rather than high-caloric environment. However, this form of metabolic memory does not seem robust, as it is vulnerably diminished under genetic or environmental influences. We postulate that this vulnerability to overnutrition is particularly prominent for mammals (such as C57BL/6J mice), and overnutritional reward-induced excess in caloric intake can quickly become dominant. This effect can be consistently induced in Drosophila when learning/memory-regulating genes are inhibited in the brain or the hypothalamus-like PI region. We observed that each of these genetic disruptions led to impaired metabolic learning, resulting in increased caloric intake and, on a chronic basis, the development of lipid excess and diabetes-like phenotype. Indeed, it has been documented that chronic high-sugar feeding is sufficient to cause insulin resistance, obesity and diabetes in Drosophila [54] , [55] . It is yet unclear whether this metabolic learning can induce an appetitive memory of normal caloric environment or an aversive memory of high-caloric environment. Regardless, our findings in this work have provoked us to raise a stimulating question, that is, whether this form of metabolic learning and memory is present in the mammals and, if so, whether this mechanism can be consolidated to improve the control of metabolic physiology and prevent against diseases. Our mouse studies in this work may provide an initial support to this concept and strategy, but clearly, in-depth future research is much needed. In light of the underlying neural basis for this metabolic learning, our study indicates that multiple brain regions are required, including the hypothalamus-like PI region in addition to the MB (equivalent to the hippocampus in mammals), which is classically needed for learning and memory formation. Anatomically, the PI region is located in the unpaired anteromedial domain of the protocerebral cortex, which is near the calyces of the MB and the dorsal part of the central complex (another brain region for regulating learning and memory) [56] . Functionally, the PI region has been demonstrated to coordinate with the MB in regulating various physiological activities in Drosophila [57] , [58] , [59] . Thus, it is very possible that some PI neurons present nutritional information to the MB and thus induce metabolic learning and memory formation. However, the underlying detailed mechanism is still unknown, especially if this process involves a role of dilps, which represent the prototypical neuropeptides produced by the PI neurons. Considering that the PI region in flies is equivalent to the mammalian hypothalamus [60] , [61] , [62] , we extended this study to mouse models by comparatively analysing A/J versus C57BL/6J mice—which are known to have different diet preference as well as different susceptibilities to obesity development [63] . We revealed that, while A/J mice showed a learning process of distinguishing NC versus HC food, C57BL/6J mice failed to do so. It is particularly notable that this difference of learning and memory between these two strains is associated with differential expression profiles of learning/memory genes in the hypothalamus rather than the hippocampus. This finding, in conjunction with our Drosophila study, highlights a potential that the hypothalamus has a unique role in mediating metabolic learning and memory formation. Although the mouse experiments cannot exclude the impacts from the taste/smell properties of the studied food, the results demonstrated that there is a form of nutritional memory, which seems dissociable from the memory of overnutritional reward. These initial observations in mice lend an agreement with our findings in Drosophila , suggesting that the brain and potentially the hypothalamus can link nutritional environment to a form of metabolic learning and memory. From a disease perspective, metabolic learning in Drosophila is impaired under chronic overnutrition, and our mouse study was in line with this understanding. This response to overnutrition is useful when famine is outstanding; however, it is a dilemma when metabolic disease is of concern, much like the scenario pertaining to leptin resistance under chronic overnutrition, whereas an increase in leptin sensitivity is demanded to reduce obesity [33] . Recently, we have established that NF-κB-dependent hypothalamic inflammation links chronic overnutrition to the central dysregulation of metabolic balance [33] . Here in this study, we showed that activation of the NF-κB pathway in the PI region weakened the function of metabolic learning and, conversely, NF-κB inhibition in this region provided a protective effect against chronic overnutrition-impaired metabolic learning. These findings are in alignment with the literature, for example, pan-neuronal NF-κB inhibition was shown to improve activity-dependent synaptic signalling and cognitive function including learning and memory formation [64] , and persistent NF-κB activation inhibits neuronal survival and the function of learning and memory formation [65] . Hence, overnutrition-induced neural NF-κB activation has a negative impact on metabolic learning and memory formation in regulating metabolic homeostasis. To summarize the findings in this work, we performed a series of behavioural studies and revealed that Drosophila have a form of metabolic learning and memory, through which the flies are directed to balance food choice with caloric intake in relevant environments. Several learning/memory-regulating genes including rut , dnc and tequila are involved in this function, and brain regions including the PI in addition to the MB are required to induce this mechanism. On the other hand, metabolic learning is impaired under chronic overnutrition through NF-κB activation, leading to excess exposure to calorie-enriched environment, which causes metabolic disorders. Overall, as elucidated in Fig. 9 , metabolic learning and memory formation by the brain and potentially the hypothalamus play a role in controlling metabolic homeostasis. Figure 9: Working model of metabolic learning and memory formation. Under an environmental condition containing normal and abnormal nutrition, Drosophila can develop a form of learning and memory of metabolic information, referred to as ‘metabolic learning & memory’, to mediate the central control of metabolic homeostasis, which requires cooperative actions of the MB and PI neurons. However, chronic overnutrition can employ NF-κB-driven neuroinflammation to impair this form of learning and memory, contributing to the development of overnutrition-induced metabolic disorders and diseases. Full size image Fly strains and culture The following transgenic and mutant flies were used: dnc 1 , rut 2080 and teq f01792 (gifts from S. Waddell, University of Massachusetts Medical School), UAS-cact (gift from S. Govind, City University of New York), and fly stocks (the Bloomington Drosophila Stock Centre) including rut 2080 ;UAS-rut + (no. 9405), elav-GAL4/cyo (no. 8765) , dilp2-GAL4/cyo (no. 37516) , 17d-GAL4 (no. 51631) , UAS-PKA inh (no. 35550) , UAS-rut RNAi (no. 27035) , UAS-dnc RNAi (no. 27250) , UAS-Rel (no. 9459) and UAS-dl (no. 9319). Canton-S flies were used as wild-type controls to dnc 1 , rut 2080 and teq f01792 . Heterozygous controls were obtained by crossing GAL4 driver or UAS effector to w1118 . All RNAi strains were generated using the VALIUM10 system, a genetic approach that has been established to induce RNAi knockdown without requiring additional introduction of dicer [25] . Flies were maintained on standard cornmeal food at 25 °C and 60% relative humidity under a 12:12-h light/dark cycle, and standard food containing 50 g l −1 yeast and a designed content of sorbitol (Sigma), which replaced sucrose, were used for the indicated experiments. Fly behaviours and phenotyping Fly olfactory conditioning test was performed according to a method adapted from the literature [66] . Briefly, a training tube containing a fly diet was supplied with an odour (OCT or MCH) as elucidated in Supplementary Fig. 1 , and odour air flow was kept constant at the speed of 15 ml s −1 . For each training cycle, 50 ∼ 100 flies were placed in a training tube with a specific food–odour combination for 24 h, and switched to a second training tube with a different food–odour combination for 24 h. The initial placement of the flies in NC or HC food was randomized. After the designed training cycles were completed, flies were subjected to preference test: following a 30-min rest in an odour-free tube, they were loaded into the odour-free middle zone of test apparatus through which flies freely chose to move into an odour-containing tube on each side. Flies were given 15 min to choose their preferred odour. The Preference Index value in each test was calculated as the number of flies that chose NC food-associated odour subtracted by the number of flies that chose high- or low-calorie food-associated odour divided by the sum of these numbers. Food intake of flies was determined using a previously established method [67] . Briefly, 10 flies per sample were fed with 2.5% blue dye-containing food for 30 min, and transferred to new tubes and homogenized in 1 ml water and filtered with 0.22-μm Millex filter. The liquid phase of homogenized samples was measured for absorbance at optical density (OD) 629 nm with spectrophotometer. Flies from the same groups without dye food were used as baseline control. Body weight of flies was measured using 10 flies per sample via an analytical balancer SI-114 (Denver Instrument). To determine fecundity, eggs were collected and counted from a vial containing 5–10 mated females over a 24-h period on day 6, and following hatching, subsequent hatched larvae were counted. These flies were fed on NC (50 g l −1 sorbitol, 50 g l −1 yeast) or a regular diet (100 g l −1 sucrose, 100 g l −1 yeast) which improves fly fecundity. Locomotive activities of flies were determined by loading them into a vial (25 mm × 95 mm) capped with foam, and flies that climbed to the top of the vials within 20 s were calculated. Procedures for lifespan assay were performed according to the literature [68] . Lifespan of flies was measured using 30 flies per vial each test, in which dead flies were recorded and live flies were transferred to new vials every other day. Fly biochemistry For TG assay, flies were homogenized in 300 μl of 0.05% PBS-Triton, and the supernatant was heated for 10 min at 70 °C to inactivate endogenous enzymes. Infinity TG Reagent (300 μl; Thermo Electron Corp) was added to 20 μl homogenate and incubated at 37 °C for 15 min. TG levels were measured as the OD value at 520 nm in Spectra Max 340 Microplate Reader and total amounts were determined using TG standard. For trehalose assay, flies were homogenized in a buffer containing 5 mM Tris pH 6.6, 137 mM NaCl and 2.7 mM KCl, followed by a heat treatment for 10 min at 70 °C to inactivate endogenous trehalase. Half of the supernatant was diluted with an equal volume of the buffer to provide the basal value, the other half was diluted with trehalase solution (Sigma) to break trehalose into free glucose at 37 °C for 20 h and glucose levels were measured using the Glucose (HK) Assay Kit (sigma) via reading of OD value at 340 nm. To measure the circulating trehalose, haemolymph was extracted by decapitation and centrifugation from 30–50 adult flies, and an aliquot of collected haemolymph was used to measure trehalose using the assay described above. Fly in situ hybridization and immunostaining Fluorescent in situ hybridization was performed using a method adapted from the literature [69] . Briefly, 500-bp DNA fragment of rutabaga -coding sequence was amplified from the wild-type drosophila cDNA using PCR and was subcloned into pBluescript II SK (Stratagene) vector. Digoxigenin (DIG) RNA-labelling mix (Roche) was used to generate DIG-labelled antisense RNA probe. Dissected brains were fixed with 4% paraformaldehyde for 20 min and were digested with proteinase K for penetration. After blocking, the brains were hybridized with a DIG-labelled probe at 65 °C overnight and incubated with anti-DIG antibody (Vector), followed by a reaction with Alexa Fluor565 secondary antibody (Invitrogen). An RNA probe with a sense probe sequence was used as the negative control. For the immunostaining, primary rat-anti-Dilp2 was used (gift from Dr Pierre Leopold at the University of Nice, France) overnight at 4 °C followed by Alexa488 anti-rat-secondary antibodies (Invitrogen). 4,6-diamidino-2-phenylindole (DAPI) staining was used to reveal all cells in the brains. Images were taken using a confocal microscope. Mouse physiology and biochemistry Eight- to ten-week-old male C57BL/6J and A/J mice purchased from the Jackson Laboratory were individually housed in a standard facility with a 12-h light cycle and 12-h dark cycle alternation. Mice were maintained on a normal chow before learning and memory experiments. HFD (Cat no. : D12451, 45% fat, 4.73 kcal g −1 ) and components/colour-matched ND (Cat no. D12450H, 10% fat, 3.85 kcal g −1 ) from Research Diets were used in the learning and memory test. Body weight of mice was measured every other day, and food intake was measured on a daily basis. Glucose tolerance test : mice were fasted overnight and then intraperitoneally injected with glucose (2 g kg −1 of body weight), and at time points 15, 30, 60 and 120 min post injection, tail vein blood glucose levels were measured with a LifeScan blood glucose-monitoring system. Serum-free fatty acid concentrations were measured using an enzymatic assay kit (Wako) according to the instruction in the manual. Mouse learning and memory of ND versus HFD was tested using a procedure adapted from the literature [24] , [49] , [50] , [51] , [52] . Briefly, each mouse was fasted for 12-h night time, and was kept for 12-h daytime alternately in a transparent cage labelled with a blue circle sign versus a green plus sign that was paired with HFD or ND. One training cycle lasted 2 days, and after the desired numbers of training cycles, preference test was performed for each mouse using a test cage containing three equal compartments divided by two walls, which were the central compartment without a sign, and two side compartments that were labelled with a blue circle sign versus a green plus sign according to the same design of the training cages. Each mouse was placed in the centre compartment for 5 min, and was then allowed to have free access to the compartments on both sides. A digital camera was used to record mouse activity and the preference to the side compartments for 15 min. The Institutional Animal Care and Use Committee of the Albert Einstein College of Medicine approved all the procedures. Quantitative PCR Total RNA was isolated using Trizol reagent (Invitrogen), and mRNA was transcribed to cDNA by using primers listed in Supplementary Table 1 and M-MLV RT System (Promega). Gene expressions were analysed using SYBR Green PCR Master Mix (Applied Biosystem). Gene expression of Drosophila and mouse samples was normalized to expression levels of RP49 and β -actin , respectively. Statistical analysis Two-tailed Student’s t -test was used for comparisons between two groups, analysis of variance and appropriate post hoc analyses were used for comparisons among more than two groups and statistical tests for each figure were justified appropriately. Sample sizes were chosen with adequate power based on the literature as well as our previous studies. Fly lifespan assay was performed using Kaplan–Meier survival analysis according to the literature [68] , and P values were determined by log-rank test. Maximum lifespan analysis was conducted on the longest-lived 10% of flies in each group. Data were presented as mean±s.e.m. P <0.05 was considered statistically significant. How to cite this article: Zhang, Y. et al. Metabolic learning and memory formation by the brain influence systemic metabolic homeostasis. Nat. Commun. 6:6704 doi: 10.1038/ncomms7704 (2015).